Correspondence: Reply to ‘Quantitative evaluation of X-ray dark-field images for microcalcification analysis in mammography’ 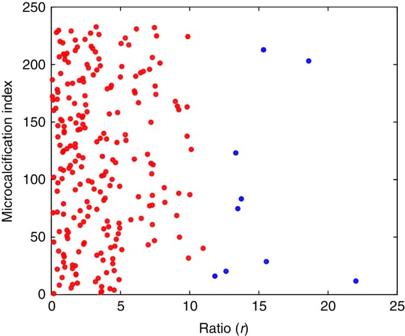Figure 1: Amended originalFig. 3d. Distribution, with rescaled R-ratio along the ascissa, of all microcalcifications visible in the specimen shown inFig. 3of the Original Article. How to cite this article : Wang Z. et al . 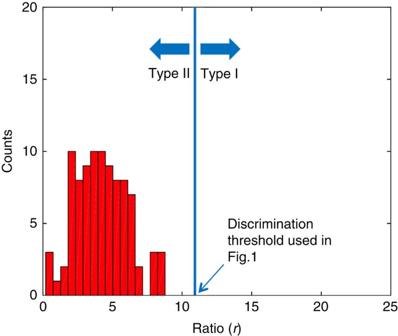Figure 2: Amended original Fig. 5f. Histogram of the ratio values of the 94 microcalcifications considered on the sample shown in Figure 5 of the original Article. The R-ratio values are distributed in the range of 0.2–9.0 around a peak value of 4.0. 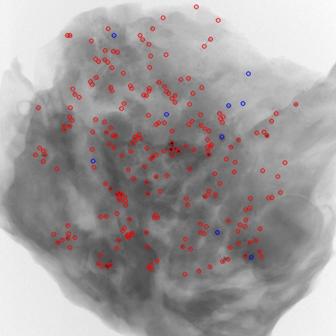Figure 3: Amended original Supplementary Fig. 1b. Classification of all microcalcifications detected in the sample shown in Figure 3 of the Original Article. The threshold was set empirically to 11, as shown in Figure 1. Accordingly, 9 Type I microcalcifications were found and marked with blue circles while 229 Type II microcalcifications were marked with red circles. Correspondence: Reply to ‘Quantitative evaluation of X-ray dark-field images for microcalcification analysis in mammography’. Nat. Commun. 7:10868 doi: 10.1038/ncomms10868 (2016).